A chloroplast envelope-bound PHD transcription factor mediates chloroplast signals to the nucleus Chloroplast development, maintenance and function depend on the coordinated expression of chloroplast and nuclear genes. The retrograde chloroplast signals are essential in coordinating nuclear gene expression. Although the sources of signals in chloroplasts have been identified and the associated transcription factors in the nucleus extensively studied, the molecular mechanism that relays chloroplast signals to the nucleus remains a mystery. Here we show that PTM, a chloroplast envelope-bound plant homeodomain (PHD) transcription factor with transmembrane domains, functions in multiple retrograde signal pathways. The proteolytic cleavage of PTM occurs in response to retrograde signals and amino-terminal PTM accumulates in the nucleus, where it activates ABI4 transcription in a PHD-dependent manner associated with histone modifications. These results provide a molecular basis for the critical function of PTM in retrograde chloroplast signaling and shed new light on the mechanism whereby chloroplast signals are transmitted to the nucleus through the cytosol. Chloroplasts have essential roles in photosynthesis and associated metabolic pathways; therefore, they are of fundamental importance for life on the Earth. The chloroplast has its own genome, which encodes only ∼ 100 genes, although more than 3,000 proteins function within the chloroplast [1] . Therefore, more than 95% of chloroplastic proteins are encoded by the nuclear genome, translated in the cytosol and post-translationally imported into the chloroplast [2] , [3] , [4] , [5] . The chloroplast-encoded and imported nuclear-encoded proteins are assembled to form functional photosynthetic and metabolic complexes [6] . Thus, tightly coordinated gene expression between the chloroplast and nuclear genomes is essential for chloroplast biogenesis and maintenance as well as for sustaining the reactions of photosynthesis. Chloroplast development and gene expression are regulated mainly by nuclear-encoded proteins, but retrograde signals from the chloroplast to the nucleus modulate the expression of nuclear genes encoding chloroplast-localized proteins to maintain the functional and metabolic states of the organelle [7] , [8] , [9] , [10] , [11] , [12] . Evidence that signals originate from chloroplasts to regulate nuclear gene expression first emerged from studies on the albostrians mutant of barley [13] . The expression of several chloroplast proteins encoded in the nucleus was reduced in mutants that had undifferentiated chloroplasts lacking ribosomes and were highly sensitive to photo-induced damage. Thus far, several chloroplast-to-nucleus retrograde signaling pathways have been identified [10] , [11] , [12] . The intermediates of tetrapyrrole biosynthesis have been implicated in the communication between the chloroplast and nucleus in both Chlamydomonas and higher plants [14] , [15] . The application of inhibitors of tetrapyrrole biosynthesis and of intermediates in tetrapyrrole biosynthesis can lead to the repression and activation of nuclear-encoded genes, respectively [16] . Further evidence was obtained through identification and characterization of gun (genome uncoupled) mutants ( gun1 through gun5 ) that block the chloroplast-to-nucleus retrograde signaling [17] . GUN2 , GUN3 , GUN4 and GUN5 encode proteins that participate in the tetrapyrrole biosynthetic pathway [15] , [18] , [19] . GUN2 , GUN3 and GUN5 encode the haem oxygenase, the phytochromobilin synthase and the H subunit of Mg-chelatase, respectively, in tetrapyrrole biosynthesis, whereas GUN4 encodes a chloroplast-localized protein that binds Proto/MgProto and regulates Mg-chelatase activity. GUN5 has also been implicated as a receptor for ABA and antagonizes a group of WRKY transcription factors to relieve the inhibition of ABA response genes, such as ABI5 , ABI4 and so on [20] , [21] . Although there are conflicting reports that the steady-state levels of Mg-protoporphyrin are not correlated to Lhcb (encoding a light-harvesting chlorophyll a/b-binding protein) expression levels [22] , [23] , the possibility exists that the rates of production and degradation of Mg-protoporphyrin function as a signal. In addition, impaired tetrapyrrole biosynthesis may cause localized generation of reactive oxygen species (ROS) or changes in the redox status of the chloroplast, which might trigger the signals [22] . The signals derived from the photosynthetic electron transfer (PET) chain seem to affect both photosynthesis-related and stress-related genes [7] , [8] , [9] . The redox state of the plastoquinone pool, other components of the photosynthetic electron transport chain and ROS are involved in the PET-derived signaling [7] , [8] , [24] , [25] , [26] , [27] . The signal is also induced by inhibition of photosynthetic gene expression (PGE) [7] , [8] , [16] . Because the gun1 mutant displays altered response to the PET-dependent, tetrapyrrole-mediated and PGE-mediated signaling pathways, it seems that multiple signal transduction pathways are integrated within the chloroplast upstream of GUN1. GUN1, a chloroplastic pentatricopeptide repeat protein co-localized with the nucleoid [28] , may either generate or transmit a second, common signal to the nucleus. The nuclear-localized APETALA2 (AP2)-type transcription factor, ABI4, was proposed to inhibit Lhcb expression by competitively binding to the G-box so as to prevent the binding of G-box transcription factors in response to GUN1-derived chloroplast signals, thus mediating the previously proposed 'master switch' [28] . However, the molecular mechanism that relays the chloroplast signals through the cytosol to the nucleus remains unknown. In this work, we show that a chloroplast envelope-bound plant homeodomain (PHD) transcription factor, designated PTM (for PHD type transcription factor with transmembrane domains), is activated by proteolytic cleavage and transmits multiple retrograde chloroplast signals to the nucleus. Functions of PTM in multiple retrograde signaling pathways The simplified signal transduction pathway raises the key question of how chloroplast signals are transmitted to the nuclear-localized ABI4 to repress nuclear gene expression. A challenging task for understanding chloroplast-to-nucleus retrograde signaling is to identify the component for transducing chloroplast signals to the nucleus. Membrane-bound transcription factors (MTFs) have been shown to regulate diverse cellular functions through an intriguing regulated proteolytic activation mechanism [29] , [30] , [31] . These MTF proteins are associated with the intracellular membranes in their dormant forms. On stimulation, they are released from the membranes through proteolytic cleavage and its cleaved MTF fragments containing the transcription factor domain are redistributed to the nucleus, where they regulate the expression of particular nuclear genes [29] , [30] , [31] . The At5g35210 gene encoding a putative chloroplast envelope-bound transcription factor PTM [31] was chosen to test its function in mediating chloroplast signals to regulate photosynthetic nuclear gene expression. To investigate the PTM functions, we analysed the retrograde response in the Arabidopsis ptm mutant carrying a transfer-DNA (T-DNA) insertion in the second exon of PTM ( Supplementary Fig. S1a–c ). Under normal growth conditions, the ptm mutant plants were indistinguishable from wild type ( Supplementary Fig. S1a ). The expression level of Lhcb in wild-type and PTM/ptm seedlings decreased by about 97% following treatment with norflurazon (NF), an inhibitor of carotenoid biosynthesis, which causes photooxidative stresses within the chloroplast in the light ( Fig. 1a ). However, treatment of ptm , gun1 and abi4 with NF resulted in a reduction in Lhcb levels to about 13%, 22%, and 15% those of the controls, respectively. NF treatment has also been shown to cause the disappearance of chloroplast ribosomes, which may indirectly trigger PGE pathway [7] . Because the signaling affected by chloroplast protein synthesis inhibitors has been shown to operate in 3-day-old seedlings [16] , we treated older seedlings with NF to exclude the potential effects of PGE. The ptm seedlings, similar to the gun1 and abi4 seedlings, were unable to repress Lhcb expression when treated with NF ( Fig. 1b ), which suggests that PTM has a role in the tetrapyrrole-mediated pathway. Treatment with plastid protein synthesis inhibitor lincomycin (Lin) also resulted in a reduction in Lhcb transcript levels, whereas the ptm seedlings, similar to the abi4 and gun1 seedlings, showed an increased accumulation of Lhcb compared with wild type ( Fig. 1c ). As NF and Lin treatments were performed in the light, it would be expected that ROS accumulate. To exclude the effects of ROS, we examined the Lhcb levels of the ptm mutant in the presence of Lin in the dark and our results showed that ptm also displayed a gun phenotype ( Supplementary Fig. S2a ), suggesting that PTM is involved in a PGE-dependent signaling pathway. 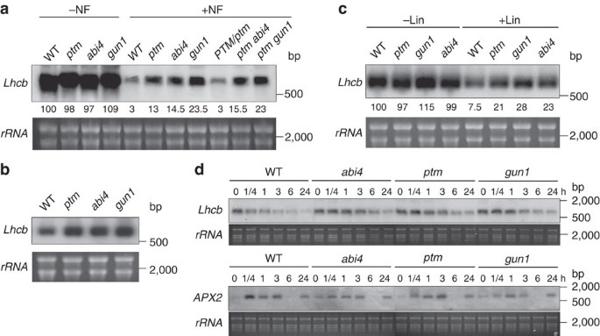Figure 1: Theptmmutant is agunmutant. (a)LhcbmRNA levels in seedlings of wild-type (WT),ptm,abi4,gun1,PTM/ptm(ptmcomplemented withPTM),ptm abi4andptm gun1mutants after treatment with norflurazon (NF).Arabidopsisseedlings were grown on 1/2 LS medium with 5 μM NF in the dark for 4 days and then transferred to light for 3 days. RNA was isolated, andLhcbmRNA levels were determined by RNA gel blot analysis. rRNA, ethidium bromide-stained ribosome RNA. (b)LhcbmRNA levels in 4-day-old green seedlings of WT,abi4,ptmandgun1mutant seedlings after treatment with NF. Four-day-oldArabidopsisseedlings grown on 1/2 LS medium were treated with 5 μM NF and collected 9 days later. (c)LhcbmRNA levels of 6-day-old seedlings of WT,ptm,abi4andgun1mutants after treatment with lincomycin (Lin).Arabidopsisseedlings were grown on 1/2 LS medium with 220 μg ml−1Lin for 6 days. (d)LhcbandAPX2mRNA levels in 4-week-old WT,abi4,ptmandgun1mutant seedlings after HL treatment. Four-week-old WT,abi4,ptmandgun1mutant seedlings grown under normal light were exposed to HL intensities for the indicated times. These experiments (a–d) were repeated three times independently, and similar results were obtained. The results from a representative experiment are shown. Figure 1: The ptm mutant is a gun mutant. ( a ) Lhcb mRNA levels in seedlings of wild-type (WT), ptm , abi4 , gun1 , PTM/ptm ( ptm complemented with PTM ), ptm abi4 and ptm gun1 mutants after treatment with norflurazon (NF). Arabidopsis seedlings were grown on 1/2 LS medium with 5 μM NF in the dark for 4 days and then transferred to light for 3 days. RNA was isolated, and Lhcb mRNA levels were determined by RNA gel blot analysis. rRNA, ethidium bromide-stained ribosome RNA. ( b ) Lhcb mRNA levels in 4-day-old green seedlings of WT, abi4 , ptm and gun1 mutant seedlings after treatment with NF. Four-day-old Arabidopsis seedlings grown on 1/2 LS medium were treated with 5 μM NF and collected 9 days later. ( c ) Lhcb mRNA levels of 6-day-old seedlings of WT, ptm , abi4 and gun1 mutants after treatment with lincomycin (Lin). Arabidopsis seedlings were grown on 1/2 LS medium with 220 μg ml −1 Lin for 6 days. ( d ) Lhcb and APX2 mRNA levels in 4-week-old WT, abi4 , ptm and gun1 mutant seedlings after HL treatment. Four-week-old WT, abi4 , ptm and gun1 mutant seedlings grown under normal light were exposed to HL intensities for the indicated times. These experiments ( a – d ) were repeated three times independently, and similar results were obtained. The results from a representative experiment are shown. Full size image We then tested whether PTM is also involved in the PET-derived signaling. Treatment with high light (HL) causes a reduction of photosynthetic electron transport chain activity and produces ROS [7] , [8] . High levels of light were effective in preventing the expression of Lhcb in wild-type seedlings, whereas decreased inhibitory effects on the expression of Lhcb were observed in ptm , gun1 and abi4 ( Fig. 1d ). We next examined the expression of APX2 (ascorbate peroxidase 2) upon exposure to HL ( Fig. 1d and Supplementary Fig. S2b ). Treatment with HL resulted in a rapid, transient accumulation of APX2 and high levels of APX2 were observed within 15 min and maintained up to 3 h in wild type. The maximal level of APX2 was observed after 1 or 3 h in gun1 , abi4 and ptm . HL is also known to be a rather complex signal that generates ROS and reduces plastoquinone pool, which may affect nuclear gene expression [7] , [8] . To distinguish these possibilities, we have examined the levels of Lhcb after treatments with dibromothymoquinone (DBMIB) (which reduce the plastiquinone pool), paraquat and rose Bengal (which would induce peroxides and singlet oxygen, respectively) under normal light conditions. The mRNA levels of Lhcb were about 3- to 4-fold higher in the ptm and gun1 mutants than wild-type plants ( Supplementary Fig. S2c ). These results suggest that PTM functions in multiple retrograde pathways. Because the above results indicate that PTM, similar to GUN1 and ABI4, has a role in multiple chloroplast-derived signals to the nucleus, we investigated the relationship between PTM, GUN1 and ABI4. To this purpose, we crossed the single mutants and obtained gun1 ptm and ptm abi4 double mutants ( Supplementary Fig. S1d–f ). Lhcb levels in gun1 ptm and abi4 ptm double mutants were similar to those in gun1 and abi4 single mutants in the presence of NF, respectively ( Fig. 1a ). Analysis of Lhcb mRNA level in N-PTM / gun1 showed that the gun1 phenotype can be suppressed by constitutive expression of N-PTM during stress ( Supplementary Fig. S2d ), which is consistent with the action of PTM downstream of GUN1. No apparent difference in the Lhcb mRNA level was observed between wild-type and transgenic plants overexpressing N-PTM in the absence of inhibitors ( Supplementary Fig. S2d ). Processing and subcellular localization of PTM during stress The PTM protein of 1,706 amino acids has amino-terminal DDT (DNA-binding homeobox and different transcription factors) [32] and PHD [33] domains with highly conserved secondary and tertiary structures and four transmembrane domains at its carboxy-terminus ( Supplementary Figs S3 and S4 ). Immunoblot analysis revealed the presence of one major band with a molecular mass of about 180 kDa, corresponding to the estimated full-length PTM, which was exclusively detected in the chloroplast outer envelope ( Fig. 2a ). Treatments with salts indicated that PTM was an intrinsic membrane protein ( Supplementary Fig. S5a ). PTM has a nuclear localization signal peptide in its N-terminus, according to the WoLF PSORT prediction [34] , and the generation of an N-terminal fragment lacking transmembrane domains but containing the complete DDT and PHD domains fused with green fluorescent protein (GFP) showed that the GFP signal was localized in the nucleus ( Fig. 2b ). Further chloroplast fractionation and immunoblot analysis showed that only one band, with a molecular weight of ∼ 58 kDa, was detected in the nuclear fraction ( Fig. 2c ). The immunoblot analysis with the antibody against the C-terminus of PTM showed that the processed form of PTM, C-PTM, was not detectable in the nucleus ( Supplementary Fig. S5b ). 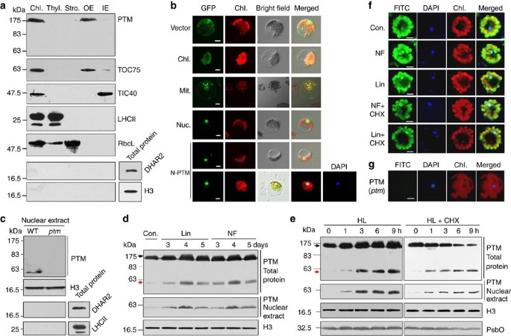Figure 2: Dual localization of PTM to the chloroplast and the nucleus. (a) Immunolocalization analysis of PTM. Intact chloroplasts (Chl.) were separated into stroma (Stro.), thylakoid membrane (Thyl.), outer envelope (OE) and inner envelope (IE) fractions. Polyclonal antibodies were used against RbcL, LHCII, TOC75, TIC40, DHAR2, Histone 3 and PTM. Sample loading was standardized by protein content (5 μg). (b) Subcellular localization of N-PTM by GFP assays. The constructs used for transformation are indicated to the left: Vector, signal of 35S::GFP vector; Chl., signal of chloroplast localization protein, RbcL; Nuc., signal of nuclear localization protein, fibrillarin; Mit., signal of mitochondrial localization protein, FRO1; N-PTM, signal from the N-PTM-GFP fusion protein. A representative image from a single protoplast is shown. Scale bar, 10 μm. (c) Nuclear localization of the processed form of PTM. The nuclear extracts from wild-type (WT) andptmplants were resolved on SDS–polyacrylamide gel electrophoresis (PAGE) followed by immunoblot analysis. (d) Effects of NF and Lin on PTM processing. Total proteins (30 μg) were isolated from the seedlings after treatments with NF and Lin, separated by SDS–PAGE and immunodetected with anti-PTM. The black arrows indicate the full-length PTM protein, and the red arrows indicate the processed form of full-length PTM. (e) Effects of high light (HL) on PTM processing. Total proteins (30 μg) were isolated from the HL-treated leaves in the presence (HL+CHX) or absence (HL) of cycloheximide, and subjected to immunoblot analysis. (f) After treatments with Lin and NF in the presence or absence of cycloheximide (CHX), the protoplasts were incubated with anti-PTM antibody followed by incubation with a secondary antibody conjugated to FITC. An untreated sample was used as a control. Scale bar, 10 μm. (g) Immunofluorescence analysis of theptmmutant with anti-PTM antibody. The 4,6-diamidino-2-phenylindole (DAPI) fluorescence, shown in blue, indicates the location of the nucleus. Chlorophyll autofluorescence was detected and shown in red. Scale bar, 10 μm. These assays (a–g) were repeated three times, and the results from a representative experiment are shown. Figure 2: Dual localization of PTM to the chloroplast and the nucleus. ( a ) Immunolocalization analysis of PTM. Intact chloroplasts (Chl.) were separated into stroma (Stro. ), thylakoid membrane (Thyl. ), outer envelope (OE) and inner envelope (IE) fractions. Polyclonal antibodies were used against RbcL, LHCII, TOC75, TIC40, DHAR2, Histone 3 and PTM. Sample loading was standardized by protein content (5 μg). ( b ) Subcellular localization of N-PTM by GFP assays. The constructs used for transformation are indicated to the left: Vector, signal of 35S::GFP vector; Chl., signal of chloroplast localization protein, RbcL; Nuc., signal of nuclear localization protein, fibrillarin; Mit., signal of mitochondrial localization protein, FRO1; N-PTM, signal from the N-PTM-GFP fusion protein. A representative image from a single protoplast is shown. Scale bar, 10 μm. ( c ) Nuclear localization of the processed form of PTM. The nuclear extracts from wild-type (WT) and ptm plants were resolved on SDS–polyacrylamide gel electrophoresis (PAGE) followed by immunoblot analysis. ( d ) Effects of NF and Lin on PTM processing. Total proteins (30 μg) were isolated from the seedlings after treatments with NF and Lin, separated by SDS–PAGE and immunodetected with anti-PTM. The black arrows indicate the full-length PTM protein, and the red arrows indicate the processed form of full-length PTM. ( e ) Effects of high light (HL) on PTM processing. Total proteins (30 μg) were isolated from the HL-treated leaves in the presence (HL+CHX) or absence (HL) of cycloheximide, and subjected to immunoblot analysis. ( f ) After treatments with Lin and NF in the presence or absence of cycloheximide (CHX), the protoplasts were incubated with anti-PTM antibody followed by incubation with a secondary antibody conjugated to FITC. An untreated sample was used as a control. Scale bar, 10 μm. ( g ) Immunofluorescence analysis of the ptm mutant with anti-PTM antibody. The 4,6-diamidino-2-phenylindole (DAPI) fluorescence, shown in blue, indicates the location of the nucleus. Chlorophyll autofluorescence was detected and shown in red. Scale bar, 10 μm. These assays ( a – g ) were repeated three times, and the results from a representative experiment are shown. Full size image It is likely that PTM is localized in the chloroplast envelope but released from the membrane by an as-yet-unidentified protease, with its cleaved MTF fragment containing the transcription factor domains being redistributed to the nucleus, where it regulates the expression of particular nuclear genes. To test this possibility, we monitored the levels of full-length PTM and its processed form after plants had been subjected to various treatments ( Fig. 2d,e ). The levels of full-length PTM increased during 4 days and decreased at day 5 after treatments with NF and Lin, and the PTM contents increased during the course of treatments with HL ( Fig. 2d,e and Supplementary Fig. S5c ). Treatments with HL, Lin and NF induced the detection of a lower band of ∼ 58 kDa, which was the same size as the N-terminal fragment without transmembrane domains (N-PTM; Fig. 2d,e ). This may in fact be the processed form of PTM, as has been reported for other MTFs [29] , [30] , [31] . In addition, immunofluorescence analysis with anti-N-PTM antibody showed that the immunofluorescence signals were predominantly detected in chloroplasts before treatment ( Fig. 2f ). After NF and Lin treatments, the shift in colour of nucleus in merged images was most obvious (pale blue with inhibitors versus dark blue in control), probably as a result of migration of processed N-terminal PTM from the chloroplast to the nucleus ( Fig. 2f ). A control experiment with the ptm mutant indicates the specificity of fluorescence signals ( Fig. 2g ). The increase in PTM levels observed in the immunoblot analysis after NF and Lin treatments was consistent with the observations that β-glucuronidase (GUS) levels and GUS activities increased after treatments with NF, and Lin in transgenic plants carrying a translational gene fusion construct PTM-GUS ( Fig. 3a–f ). 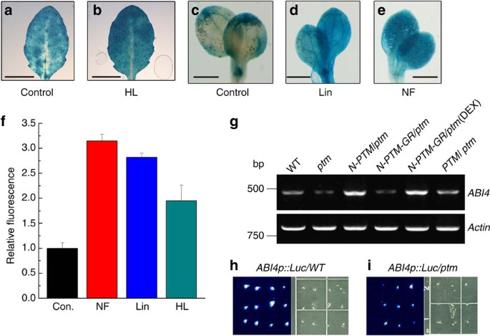Figure 3: Expression ofPTMp::PTM-GUSandABI4. (a) The GUS staining of the transgenicPTM-GUSleaves. Scale bar, 5 mm. (b) The GUS staining of the transgenicPTM-GUSleaves after treatment with high light (HL; 1 h). Scale bar, 5 mm. (c) The GUS staining of the transgenicPTM-GUSseedling cotyledon. Scale bar, 0.5 mm. (d,e) The GUS staining of the transgenicPTM-GUSseedling cotyledon after treatments with norflurazon (NF, 5 days) and lincomycin (Lin, 5 days), respectively. Scale bar, 0.5 mm. (f) The GUS activities of the transgenicPTM-GUSseedling cotyledon after treatments with NF (5 days), Lin (5 days) or leaves after treatments with HL (1 h). Values are means of triplicate measurements with error bars representing the standard deviation. (g) Expression ofABI4in wild type (WT),ptm, N-PTM/ptm,PTM/ptmandN-PTM-GR/ptm. Six-day-old WT,ptm, PTM/ptm, N-PTM/ptmandN-PTM-GR/ptmseedlings were grown in 1/2 LS media used for RT–PCR (dexamethasone (DEX) indicates seedlings were grown in 1/2 LS media with 1 μM DEX). PCR amplification was performed usingABI4primers.Actinwas used as a control. (h,i) Luminescence in the transgenicABI4p::Luc/WT (h) andABI4p::Luc/ptm(i) lines. These experiments (a–eandg–i) were repeated three times independently, and similar results were obtained. The results from a representative experiment are shown. Figure 3: Expression of PTMp::PTM-GUS and ABI4 . ( a ) The GUS staining of the transgenic PTM-GUS leaves. Scale bar, 5 mm. ( b ) The GUS staining of the transgenic PTM-GUS leaves after treatment with high light (HL; 1 h). Scale bar, 5 mm. ( c ) The GUS staining of the transgenic PTM-GUS seedling cotyledon. Scale bar, 0.5 mm. ( d , e ) The GUS staining of the transgenic PTM-GUS seedling cotyledon after treatments with norflurazon (NF, 5 days) and lincomycin (Lin, 5 days), respectively. Scale bar, 0.5 mm. ( f ) The GUS activities of the transgenic PTM-GUS seedling cotyledon after treatments with NF (5 days), Lin (5 days) or leaves after treatments with HL (1 h). Values are means of triplicate measurements with error bars representing the standard deviation. ( g ) Expression of ABI4 in wild type (WT), ptm, N-PTM/ptm , PTM/ptm and N-PTM-GR/ptm . Six-day-old WT, ptm, PTM/ptm, N-PTM/ptm and N-PTM-GR/ptm seedlings were grown in 1/2 LS media used for RT–PCR (dexamethasone (DEX) indicates seedlings were grown in 1/2 LS media with 1 μM DEX). PCR amplification was performed using ABI4 primers. Actin was used as a control. ( h , i ) Luminescence in the transgenic ABI4p::Luc/ WT ( h ) and ABI4p::Luc / ptm ( i ) lines. These experiments ( a – e and g – i ) were repeated three times independently, and similar results were obtained. The results from a representative experiment are shown. Full size image To examine whether N-PTM was derived from full-length PTM, the leaves were treated with cycloheximide (CHX) under HL. The nuclear-encoded PsbO protein levels were decreased gradually in the presence of CHX, but remained almost unchanged in the absence of CHX ( Fig. 2e ), which indicates that CHX can efficiently inhibit nuclear-encoded protein synthesis. The full-length PTM protein contents were decreased in the presence of CHX ( Fig. 2e ) because of reduced protein synthesis and continued PTM degradation. The levels of N-PTM increased gradually after HL treatment in the presence of CHX. Examination of the processing and localization of PTM in the gun1 mutant showed that the levels of full-length PTM and processed N-PTM were decreased during stress ( Supplementary Fig. S5c ), which suggests that GUN1 is important for increased PTM expression during stress. In addition, immunofluorescence analysis with anti-N-PTM antibody showed that the immunofluorescence signals in the chloroplasts were decreased after treatments with NF and Lin in the presence of CHX, whereas the signals in the nucleus were increased ( Fig. 2f ). These results indicate that N-PTM was processed from full-length PTM. As shown in Supplementary Figure S5d , PTM processing was dramatically suppressed by serine protease inhibitor pefabloc, but not by aspartic protease inhibitor pepstatin. Further examination of the cleavage of PTM in isolated chloroplasts treated with Lin showed that PTM contents were decreased gradually in the absence of pefabloc, but the levels of PTM remained relatively stable in the presence of pefabloc. These results indicated that PTM can be processed by the protease in the envelope ( Supplementary Fig. S5e ). Transcriptional activation activity of PTM Semi-quantitative reverse transcription PCR (qRT–PCR) analysis showed that ABI4 expression was reduced in the ptm mutant, and the level of ABI4 was restored in the ptm- complemented line ( Fig. 3g ). The effect of PTM on ABI4 expression was further examined by crossing ptm with plants carrying the luciferase reporter gene fused to the ABI4 promoter ( ABI4p::Luc ). The luminescence intensities in the ptm seedlings were considerably lower than those in wild type ( Fig. 3h,i ). These results indicate that PTM is required for the proper expression of ABI4 . We further generated transgenic plants expressing N-PTM proteins fused with a glucocorticoid receptor (GR) to control nuclear localization and our results showed that the expression of ABI4 was recovered in N-PTM-GR / ptm only in the presence of 1 μM dexamethasone but not in its absence ( Fig. 3g ). These results indicate that the nuclear localization of PTM is required for normal ABI4 expression. Next we examined whether the ptm mutant showed ABA resistant. Our results showed that gun1 and ptm appeared intermediate between wild type and abi4 in germination assays, which suggests the possible function of PTM in ABA signaling ( Supplementary Fig. S6 ). We next performed a chromatin immunoprecipitation (ChIP) assay to examine whether processed PTM binds to the promoter region of ABI4 . Multiplex PCR revealed that fragment ABI4p-4 (−288/−20) was enriched in the ABI4 promoter in the anti-PTM samples compared with the ChIP samples prepared with preimmune antisera and actin controls ( Fig. 4a,b ). We next used a yeast one-hybrid assay to delineate the DNA sequences to which N-PTM binds. Gal4 transcriptional activation domain N-PTM (GAD-N-PTM) fusion proteins, but not GAD alone, activated the LacZ reporter genes driven by fragment ABI4p-4 , but not fragments ABI4p1-3 of ABI4 promoters, which provided further support for these findings ( Fig. 4c ). These results suggest that PTM is associated with the ABI4 promoter in vivo . 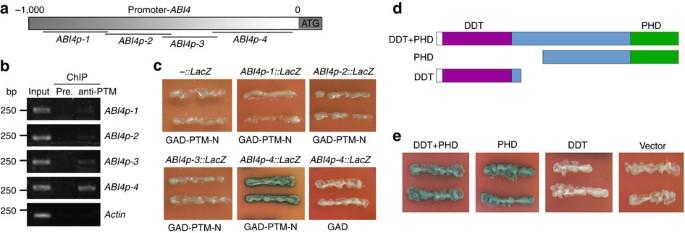Figure 4: PTM binds directly to the promoter ofABI4. (a) Diagram of the promoter fragments ofABI4. The locations of PCR primers (ABI4p-1,ABI4p-2,ABI4p-3andABI4p-4) used for the enrichment test are indicated, and the numbers indicate base pairs relative to the initiation site, which is indicated by '0'. (b) PTM binds directly toABI4promoter. ChIP analysis was performed using N-PTM antibody, and genomic DNA obtained by ChIP was subjected to PCR analysis. Immunoprecipitation with a preimmune (Pre.) sample was used as a control. The PCR fragmentsABI4p-1,ABI4p-2,ABI4p-3andABI4p-4represent four fragments ofABI4promoter, which were shown ina. (c) PTM can activate expression of theLacZreporter gene driven by theABI4p-4::LacZin yeast. The plasmids GAD-N-PTM with–::LacZ,ABI4p-1::LacZ,ABI4p-2::LacZ,ABI4p-3::LacZandABI4p-4::LacZ; and GAD itself, withABI4p-4::LacZ, were co-transformed into the yeast strain EGY48. Transformants were grown on proper dropout plates containing X-gal (5-bromo-4-chloro-3-indolyl-β-D-galactopyranoside) for blue colour development. (d) Diagram of PTM constructs (all fused with GAD) used in the yeast one-hybrid assay. The N-terminal PHD finger motif and the DDT domain are shown. (e) Yeast one-hybrid assay showing that the N-terminal fragments of PTM (containing the DDT and PHD domain) and PHD domain alone can activate theABI4p::LacZreporter gene expression. Similar results (a–e) were obtained in two additional independent experiments. Figure 4: PTM binds directly to the promoter of ABI4 . ( a ) Diagram of the promoter fragments of ABI4 . The locations of PCR primers ( ABI4p-1 , ABI4p-2 , ABI4p-3 and ABI4p-4 ) used for the enrichment test are indicated, and the numbers indicate base pairs relative to the initiation site, which is indicated by '0'. ( b ) PTM binds directly to ABI4 promoter. ChIP analysis was performed using N-PTM antibody, and genomic DNA obtained by ChIP was subjected to PCR analysis. Immunoprecipitation with a preimmune (Pre.) sample was used as a control. The PCR fragments ABI4p-1 , ABI4p-2 , ABI4p-3 and ABI4p-4 represent four fragments of ABI4 promoter, which were shown in a . ( c ) PTM can activate expression of the LacZ reporter gene driven by the ABI4p-4::LacZ in yeast. The plasmids GAD-N-PTM with –::LacZ , ABI4p-1::LacZ , ABI4p-2::LacZ , ABI4p-3::LacZ and ABI4p-4::LacZ ; and GAD itself, with ABI4p-4::LacZ , were co-transformed into the yeast strain EGY48. Transformants were grown on proper dropout plates containing X-gal (5-bromo-4-chloro-3-indolyl-β- D -galactopyranoside) for blue colour development. ( d ) Diagram of PTM constructs (all fused with GAD) used in the yeast one-hybrid assay. The N-terminal PHD finger motif and the DDT domain are shown. ( e ) Yeast one-hybrid assay showing that the N-terminal fragments of PTM (containing the DDT and PHD domain) and PHD domain alone can activate the ABI4p::LacZ reporter gene expression. Similar results ( a – e ) were obtained in two additional independent experiments. Full size image Domain deletion analysis revealed that the portion of the N-terminal fragments containing PHD domains are necessary and sufficient for activating LacZ reporter genes driven by the ABI4 promoter ( Fig. 4d,e ). To test whether PTM has an intrinsic transcriptional regulatory activity, we fused PTM and N-PTM (the N-terminus, containing complete DDT and PHD domains) with Gal4 DNA-binding domain. The pGBK-N-PTM fusion protein, but not the pGBK-PTM, activated transcription of reporter genes HIS3 and MEL1, which were driven by the Gal4 operator ( Fig. 5a ). Immunoblot analysis showed the expression of N-PTM, N-PTM mutants and PTM in the nucleus of yeast ( Fig. 5b,c ). This result suggests that the processing of PTM is necessary for its function. In addition, mutations of critical cysteine residues at positions 426 and 429 to alanines in the pGBK-N-PTM fusion protein failed to activate transcription of reporter genes HIS3 and MEL1 ( Fig. 5a ). Indeed, mutation analysis has also revealed the importance of corresponding cysteine residues in PHD domain for transcriptional activity [33] , [35] , and substitution of cysteine residue with alanine in the PHD core region N-PTM (C429A) reduced the transcriptional activity, however, substitutions of other cysteine or histidine residues with alanine (N-PTM (C414A), N-PTM (C417A), N-PTM (C426A), N-PTM (H434A), N-PTM (H434A, C437A) and N-PTM (C452A, C455A)) had no effect. These results indicate that the 426C and 429C residues are necessary for transcription activation. In addition, PTM, but not C426A/C429A mutant protein, activated a luciferase reporter gene driven by the ABI4 promoter in Arabidopsis protoplasts ( Fig. 5d ). These results suggest that the PHD domain is essential for transcriptional activation activity and that C426 and C429 residues are important for PTM function. 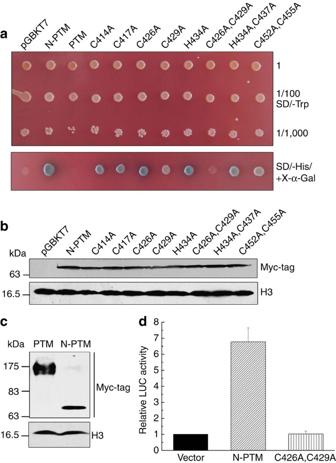Figure 5: PTM has an intrinsic transcription activation activity. (a) pGBK-N-PTM, N-PTM (C414A), N-PTM (C417A), N-PTM (C426A), N-PTM (C429A), N-PTM (H434A), N-PTM (H434A, C437A) and N-PTM (C452A, C455A) fusion proteins activateHISandMELreporter gene expression in yeast Y2HGold, whereas pGBKT7 alone, pGBK-PTM and N-PTM (C426A, C429A) fail to activate reporter gene expression. Similar results were obtained in two additional independent experiments. The results from a representative experiment are shown. (b) Immunoblot analysis of the N-PTM and N-PTM mutant proteins in the yeast nucleus. The nuclear proteins of yeast were isolated, separated by SDS–polyacrylamide gel electrophoresis, and immunodetected with anti-Myc-tag (the c-Myc epitope tag in the vector pGBKT7). The anti-H3 antibody was used as a control. (c) Immunoblot analysis with anti-Myc-tag showing the location of PTM and N-PTM in the yeast nucleus. (d) Wild-type pBSK-35S::N-PTM, but not pBSK-35S::N-PTM(C426A, C429A) or pBSK-35Sitself, activatesABI4p::Lucreporter gene expression inArabidopsisprotoplasts. Error bars represent s.d. values of triplicate experiments. LUC, luciferase. Figure 5: PTM has an intrinsic transcription activation activity. ( a ) pGBK-N-PTM, N-PTM (C414A), N-PTM (C417A), N-PTM (C426A), N-PTM (C429A), N-PTM (H434A), N-PTM (H434A, C437A) and N-PTM (C452A, C455A) fusion proteins activate HIS and MEL reporter gene expression in yeast Y2HGold, whereas pGBKT7 alone, pGBK-PTM and N-PTM (C426A, C429A) fail to activate reporter gene expression. Similar results were obtained in two additional independent experiments. The results from a representative experiment are shown. ( b ) Immunoblot analysis of the N-PTM and N-PTM mutant proteins in the yeast nucleus. The nuclear proteins of yeast were isolated, separated by SDS–polyacrylamide gel electrophoresis, and immunodetected with anti-Myc-tag (the c-Myc epitope tag in the vector pGBKT7). The anti-H3 antibody was used as a control. ( c ) Immunoblot analysis with anti-Myc-tag showing the location of PTM and N-PTM in the yeast nucleus. ( d ) Wild-type pBSK- 35S::N-PTM , but not pBSK- 35S::N-PTM ( C426A, C429A ) or pBSK- 35S itself, activates ABI4p::Luc reporter gene expression in Arabidopsis protoplasts. Error bars represent s.d. values of triplicate experiments. LUC, luciferase. Full size image PTM binding and histone modification during stress A subset of PHD domains, including ING2 and ORC1, have been shown to interact with methylated histones [35] , [36] . Mutational analyses of human ING2 and Arabidopsis ORC1b PHD motif have demonstrated that residue W238 or G188 is part of the cage that contributes to the interaction with H3K4me3 [35] , [36] , [37] . Residues D412, G421 and L423 of PTM are highly conserved in the equivalent positions ( Fig. 6a ). To investigate the functional relevance of the PHD domain of PTM, we first assessed its interaction with biotinylated histones. PTM was able to pull-down H3K4me3, whereas binding of PTM to unmodified histones H3, H3K9me3 or H4K20me3 was not detectable ( Fig. 6b ). Mutations of two cysteine residues of PTM-PHD to alanines (C426A, C429A) reduced, but did not completely abolish, the interaction of PTM-PHD with H3K4me3. Mutations of the D412, G421 and L423 residues of PTM revealed their importance for H3K4me3 binding, although residual binding was still detectable ( Fig. 6b ). 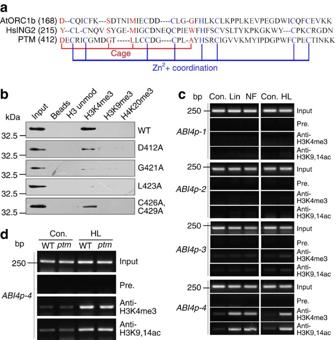Figure 6: Histone modifications in the promoter ofABI4. (a) The main cysteine (C) and histidine (H) residues of PHD regions appear in blue, and aspartic (D), glycine (G), leucine (L) and alanine (A) residues of the cage are in red. The key C and H residues of the Zn2+fingers, and the D, G, L residues of the cage that were mutated in this study are shown. (b) PTM specifically interacts with H3K4me3. Pull-down assays of biotinylated native H3 unmod., H3K4me3, H3K9me3 and H4K20me3 peptides by GST-PTM-PHD and various mutations of GST-PTM-PHD (D412A, G421A, L423A, C426A/C429A) are shown. Bound proteins were detected by immunoblot analysis with anti-GST. (c) The levels of H3K4me3 and H3K9,14ac were increased in the promoter ofABI4after NF, LIN and HL treatments for 6 h. ChIP assays were performed with anti-H3K4me3 and anti-H3K9,14ac antibodies withArabidopsischromatin. The samples were analysed by PCR using primers that matched selected fragments ofABI4p-1,ABI4p-2,ABI4p-3andABI4p-4. The samples were treated as described in fig1a,c,d. The untreated samples were used as control. (d) ChIP analyses of the levels of H3K4me3 and H3K9,14ac in the promoter of ABI4 after HL treatment. After wild-type (WT) andptmmutant plants were treated by HL for 6 h, ChIP assays were performed with anti-H3K4me3 and anti-H3K9,14ac antibodies with WT andptmmutant chromatin. The samples were analysed by PCR using primers that matched selected fragment ofABI4p-4. The untreated samples were used as controls. These experiments (b–d) were repeated three times independently, and similar results were obtained. The results from a representative experiment are shown. Con. control; Pre., preimmune. Figure 6: Histone modifications in the promoter of ABI4 . ( a ) The main cysteine (C) and histidine (H) residues of PHD regions appear in blue, and aspartic (D), glycine (G), leucine (L) and alanine (A) residues of the cage are in red. The key C and H residues of the Zn 2+ fingers, and the D, G, L residues of the cage that were mutated in this study are shown. ( b ) PTM specifically interacts with H3K4me3. Pull-down assays of biotinylated native H3 unmod., H3K4me3, H3K9me3 and H4K20me3 peptides by GST-PTM-PHD and various mutations of GST-PTM-PHD (D412A, G421A, L423A, C426A/C429A) are shown. Bound proteins were detected by immunoblot analysis with anti-GST. ( c ) The levels of H3K4me3 and H3K9,14ac were increased in the promoter of ABI4 after NF, LIN and HL treatments for 6 h. ChIP assays were performed with anti-H3K4me3 and anti-H3K9,14ac antibodies with Arabidopsis chromatin. The samples were analysed by PCR using primers that matched selected fragments of ABI4p-1 , ABI4p-2 , ABI4p-3 and ABI4p-4 . The samples were treated as described in fig 1a,c,d . The untreated samples were used as control. ( d ) ChIP analyses of the levels of H3K4me3 and H3K9,14ac in the promoter of ABI4 after HL treatment. After wild-type (WT) and ptm mutant plants were treated by HL for 6 h, ChIP assays were performed with anti-H3K4me3 and anti-H3K9,14ac antibodies with WT and ptm mutant chromatin. The samples were analysed by PCR using primers that matched selected fragment of ABI4p-4 . The untreated samples were used as controls. These experiments ( b – d ) were repeated three times independently, and similar results were obtained. The results from a representative experiment are shown. Con. control; Pre., preimmune. Full size image The histone methylation and acetylation status were associated with gene transcriptional activity [35] , [36] , [37] , [38] , [39] . ChIP assays showed that H3K4me3 increased in fragment ABI4p-4 (−288/−20) of the ABI4 promoter when the plants were treated with NF, Lin or HL. Further examination of the acetylation status of PTM-bound region of ABI4 promoter revealed that H3K9,14 acetylation increased after treatments with NF, Lin or HL ( Fig. 6c ). However, HL-induced increase in H3K4me3 and H3K9,14ac was retained in ptm , which suggests that PTM is not required for histone modifications ( Fig. 6d ). PTM activation associated with ABI4 and Lhcb gene expression We next monitored the ABI4 and PTM expression during retrograde responses by transforming Arabidopsis plants with ABI4p::Luc and PTMp::Luc . The activities of PTMp::Luc showed a very similar pattern to that of ABI4p::Luc , and the LUC activities of both PTMp::Luc and ABI4p::Luc were increased after HL treatment ( Supplementary Fig. S7a,b ). The LUC activities of both PTMp::Luc and ABI4p::Luc increased with the duration of treatments up to 4 days, and LUC activities decreased after treatment for 5 days in the presence of Lin or NF ( Supplementary Fig. S7c,d ). To determine whether the reporter gene expression was the causation of a change in mRNA levels, we examined the levels of both ABI4 and PTM with qRT–PCR. Similar results to the changes of LUC activities in response to retrograde signal were obtained (compare Fig. 7a,b with Supplementary Fig. S7a,b ; compare Fig. 7c,d with Supplementary Fig. S7c,d ). Genevestigator microarray data also showed that ABI4 expression is induced by environmental stresses, such as high temperature, HL, cold, salt stress and so on [40] . These results indicate that induction of ABI4 expression may be important for its function in chloroplast-to-nucleus signaling. 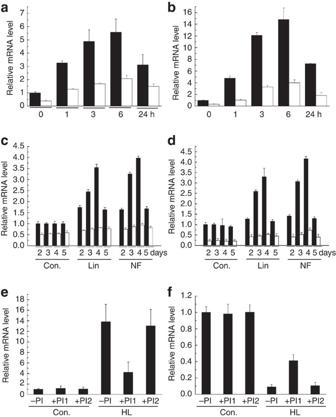Figure 7: Activation ofABI4gene expression by PTM. (a) Expression ofPTMin WT andgun1after HL treatment. After treatment with HL for various numbers of hours, RNA was extracted and the level ofPTMmRNA was analysed by qRT–PCR. Black and white bars indicate wild type (WT) andgun1, respectively. (b) Expression ofABI4in WT andgun1after HL treatment. After treatments with HL for various numbers of hours, RNA was extracted and the level ofABI4mRNA was analysed by qRT–PCR. Black and white bars indicate WT andgun1, respectively. (c) Expression ofPTMin WT andgun1after treatments with NF and Lin. WT andgun1mutant seedlings were grown in media in the presence of Lin and NF and collected after various numbers of days. After treatments, RNA was extracted and the level ofPTMmRNA was analysed by qRT–PCR. Black and white bars indicate WT andgun1, respectively. (d) Expression ofABI4in WT andgun1after treatments with NF and Lin. WT andgun1seedlings were grown in media in the presence of Lin and NF, and collected after various numbers of days. After treatments, RNA was extracted and the level ofABI4mRNA was analysed by qRT–PCR. Black and white bars indicate WT andgun1, respectively. (e) Transcript levels ofABI4in the presence of protease inhibitors under HL. After treatments with HL in the presence of pefabloc (+PI1) and pepstatin (+PI2) or absence of protease inhibitors (−IP) for 6 h, RNA was extracted, and the level ofABI4mRNA was analysed by qRT–PCR. The samples without HL treatment were used as control (Con.). (f) Transcript levels ofLhcbin the presence of protease inhibitors under HL. After treatments with HL in the presence of pefabloc (+PI1) and pepstatin (+PI2) or absence of protease inhibitors (−IP) for 6 h, RNA was extracted and the level ofABI4mRNA was analysed by qRT-PCR. The samples without HL treatment were used as control (Con.). Values are means of triplicate measurements with error bars representing the standard deviation. Figure 7: Activation of ABI4 gene expression by PTM. ( a ) Expression of PTM in WT and gun1 after HL treatment. After treatment with HL for various numbers of hours, RNA was extracted and the level of PTM mRNA was analysed by qRT–PCR. Black and white bars indicate wild type (WT) and gun1 , respectively. ( b ) Expression of ABI4 in WT and gun1 after HL treatment. After treatments with HL for various numbers of hours, RNA was extracted and the level of ABI4 mRNA was analysed by qRT–PCR. Black and white bars indicate WT and gun1 , respectively. ( c ) Expression of PTM in WT and gun1 after treatments with NF and Lin. WT and gun1 mutant seedlings were grown in media in the presence of Lin and NF and collected after various numbers of days. After treatments, RNA was extracted and the level of PTM mRNA was analysed by qRT–PCR. Black and white bars indicate WT and gun1 , respectively. ( d ) Expression of ABI4 in WT and gun1 after treatments with NF and Lin. WT and gun1 seedlings were grown in media in the presence of Lin and NF, and collected after various numbers of days. After treatments, RNA was extracted and the level of ABI4 mRNA was analysed by qRT–PCR. Black and white bars indicate WT and gun1 , respectively. ( e ) Transcript levels of ABI4 in the presence of protease inhibitors under HL. After treatments with HL in the presence of pefabloc (+PI1) and pepstatin (+PI2) or absence of protease inhibitors (−IP) for 6 h, RNA was extracted, and the level of ABI4 mRNA was analysed by qRT–PCR. The samples without HL treatment were used as control (Con.). ( f ) Transcript levels of Lhcb in the presence of protease inhibitors under HL. After treatments with HL in the presence of pefabloc (+PI1) and pepstatin (+PI2) or absence of protease inhibitors (−IP) for 6 h, RNA was extracted and the level of ABI4 mRNA was analysed by qRT-PCR. The samples without HL treatment were used as control (Con.). Values are means of triplicate measurements with error bars representing the standard deviation. Full size image We further elucidated the role of PTM processing in regulating Lhcb expression in response to retrograde signals under HL by treating leaves with protease inhibitor to block PTM processing. Under HL, qRT–PCR analysis showed that the level of ABI4 was increased by about 14- and 4-fold, respectively, in the absence and presence of protease inhibitor pefabloc ( Fig. 7e ). Treatment with pepstatin had no inhibitory effect on ABI4 expression under HL ( Fig. 7e ). Lhcb level was decreased by about 90% after treatments with HL in the absence of protease inhibitors or in the presence of pepstain. However, the level of Lhcb was about 40% of the controls after HL treatment in the presence of pefabloc ( Fig. 7f ). Similar results to the changes of LUC activities in response to retrograde signals during HL treatment were obtained (compare Fig. 7e,f with Supplementary Fig. S7e,f ). These results suggest that the processing of PTM is important for mediating chloroplast signals to the nucleus. We have demonstrated here for the first time, to our knowledge, that regulated intramembrane proteolysis is involved in regulating retrograde chloroplast-to-nucleus signaling. The dormant PTM is associated with chloroplast envelope, while only processed form of PTM was detected in nucleus, where it activates ABI4 transcription in a PHD-dependent manner ( Fig. 8 ). Transcriptional regulation of gene expression depends on the reading of histone post-translational modifications [35] . The PHD finger has been identified as a bona fide 'reader' domain because PHD fingers recognize histone post-translational modifications. Our results show that PTM contains a functional PHD domain that interacts with H3K4me3 ( Fig. 6 ). The interaction between H3K4me3 and proteins containing a PHD is ultimately coupled to changes in the histone acetylation and/or methylation statuses that are responsible for transcriptional regulation [37] , [38] , [39] . PTM-dependent transcription activation is associated with an increase in the acetylation of H3k9,14 and trimethylation of H3K4 in response to treatments with NF, Lin and HL ( Fig. 6 ). Thus, our results indicate that PTM is a H3K4me3 effector protein and that activation of ABI4 gene expression is mediated by binding of a functional domain to the ABI4 promoter. 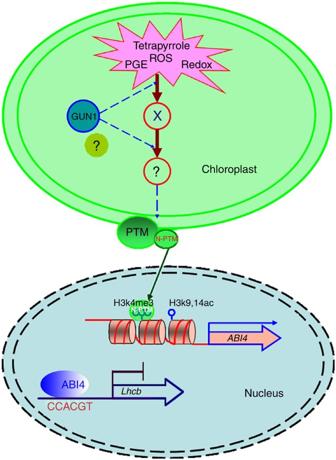Figure 8: A model showing that PTM acts as a sensor/transducer in the retrograde signaling pathways from chloroplasts. When plastid development is impaired or when plastids are stressed, inhibition of PGE, perturbation of tetrapyrrole biosynthesis, production of ROS and changes in the redox state of PET generate chloroplast retrograde signals. These signals converge on GUN1, which either generates or transmits a second signal. X could either be a process facilitated by GUN1 or a product of GUN1 activity. Unknown steps in the pathway are indicated by question marks. In response to chloroplast signals, PTM is processed into a mature form, which is redistributed to the nucleus, where it binds to the promoter ofABI4. Activation ofABI4expression was associated with histone modifications. Figure 8: A model showing that PTM acts as a sensor/transducer in the retrograde signaling pathways from chloroplasts. When plastid development is impaired or when plastids are stressed, inhibition of PGE, perturbation of tetrapyrrole biosynthesis, production of ROS and changes in the redox state of PET generate chloroplast retrograde signals. These signals converge on GUN1, which either generates or transmits a second signal. X could either be a process facilitated by GUN1 or a product of GUN1 activity. Unknown steps in the pathway are indicated by question marks. In response to chloroplast signals, PTM is processed into a mature form, which is redistributed to the nucleus, where it binds to the promoter of ABI4 . Activation of ABI4 expression was associated with histone modifications. Full size image PTM seems to participate in multiple chloroplast signals because the expression of Lhcb was uncoupled during various treatments ( Figs 1 and 8 ). ABI4 expression levels were elevated in response to treatments with Lin, NF and HL ( Fig. 7 ). In addition, expression of PTM and ABI4 showed similar patterns during treatments with NF, Lin and HL ( Fig. 7 and Supplementary Fig. S7 ). Treatment with HL in the presence of perfabloc, which inhibited the processing of PTM, not only lowered the increasing extent of ABI4 expression but also resulted in the derepression of Lhcb expression ( Fig. 7f ). Taken together, these results demonstrate the role of PTM processing in the activation of ABI4 , which is important for the suppression of Lhcb during the retrograde signaling. Our results support a model for the critical function of PTM in mediating signals from damaged and undeveloped chloroplasts to the nucleus ( Fig. 8 ). However, transgenic plants overexpressing the processed PTM did not induce a retrograde response in the absence of inhibitors ( Supplementary Fig. S2d ). Perhaps an additional signal mediated by GUN1 is also required. Woodson et al . [41] reported that haem can act as a positive signaling molecular regulating the photosynthetic-associated nuclear expression. Haem is likely to be responsible for the positive regulation of the photosynthetic-associated nuclear gene expression. There may be possible for a role of Proto/MgProto in this process. How tetrapyrroles may influence PTM and its ability to signal appears to be still an open question. These results provide a molecular basis for the critical function of PTM in mediating signals from chloroplasts to the nucleus and shed new light on the mechanism whereby the chloroplast signals are transmitted to the nucleus through the cytosol. Genes for PTM homologs exist in the nuclear genomes of plant species ( Supplementary Fig. S3 ). All PTM proteins share conserved DDT and PHD domains at their N-terminus and four transmembrane domains at their C-terminus, which suggests an evolutionarily conserved mechanism for retrograde chloroplast signaling in higher plants. However, such mechanism is unlikely to exist in Chlamydomonas because no homologous protein to PTM was found. The chloroplast localization of PTM places it an ideal place to initiate rapid transcriptional responses to developmental and functional states of chloroplasts. As chloroplasts serve as the sensors of changes in growth environment, such communication could be important in establishing proper balance of gene expression allowing plants to respond to stressful environment. Future analysis regarding how PTM senses retrograde signals within the chloroplast, how dormant PTM transcription factor is activated, and how PTM works in this complex signaling network will be of great interest in understanding cell signaling in plants and will lead to a further understanding of the role of chloroplast retrograde signaling in plant growth and development. Plant materials and growth conditions The following Arabidopsis thaliana mutants in the Columbia ecotype were obtained from the Arabidopsis Biological Resource Center: abi4 ( abi4-1 , an X-ray mutant (CS8104)), gun1 (SAIL_742_A11, a T-DNA insertion mutant) and ptm (SALK_013123, a T-DNA insertion mutant). The T-DNA insertion homozygous lines were confirmed by PCR using the following gene-specific and T-DNA-specific primers: PTMLP , PTMRP , and T-DNA LB for PTM ; and GUN1LP , GUN1RP , and T-DNA LB for GUN1 . The DNA fragments around the sites of T-DNA insertions were amplified and cloned into the plasmid vector pGEM-T (Promega), and the precise location of T-DNA insertion was determined by sequencing. Plants homozygous for the T-DNA insertions (identified by PCR analyses) were obtained, and single mutants were backcrossed to wild-type plants three times before generating double mutants to segregate out additional mutations. All of the mutants and wild-type plants were grown in growth chambers at 22 °C and 120 μmol m −2 s −1 with a 10-h-light and 14-h-dark photoperiod. For NF and Lin treatments, the mutant and wild-type seeds were surface-sterilized and plated on 1/2 Linsmaier and Skoog (1/2 LS) medium (PhytoTechnology Laboratories, LLC) containing 2% sucrose and 0.8% agar with either 5 μM NF (Sandoz Pharmaceuticals) or 220 μg ml −1 Lin (Sigma). For HL treatments, seedlings grown for 4 weeks under normal light conditions were exposed to HL (1,800 μmol m −2 s −1 ) for various lengths of time. Northern blots analysis RNA was extracted with the RNeasy kit (Qiagen). For northern blot analysis, total RNA isolated from the wild-type and mutant plants was fractionated, transferred onto nylon membranes, and subsequently probed with [32] P-labeled complementary DNA probes. Semi-quantitative and quantitative RT–PCR For semi-quantitative RT–PCR, total RNA was treated with RNase-free DNase I (Takara) to remove genomic DNA before first-strand cDNA synthesis. First-strand cDNA was generated using the PrimeScript II 1st Strand cDNA Synthesis Kit (Takara), and PCR analysis was performed with gene-specific primers using the first-strand cDNA as a template. For quantitative real-time RT–PCR, the RNA samples were reverse transcribed into first-strand cDNA using a PrimeScript RT reagent Kit (Takara). PCR was then carried out using gene-specific primers and SYBR Premix ExTaq reagent (Takara) with an Mx3000p Real-time PCR System (Agilent, Stratagene) following the manufacturer's instructions. PCR reactions were performed in triplicate for each sample, and the expression levels were normalized to an actin gene. Yeast transcription activity For the transcription activity assay, pGBKT7, pGBK-N-PTM, N-PTM(C426A,C429A), N-PTM(C414A), N-PTM(C417A), N-PTM(C426A), N-PTM(C429A), N-PTM(H434A), N-PTM(H434A,C437A) and N-PTM(C452A,C455A) were transformed into Y2HGold yeast cells and streaked on synthetic dropout nutrient medium (SD/-Trp) or (SD/-His) containing X-α-Gal agar plates. Yeast one-hybrid assay The plasmid GAD-N-PTM, with —::LacZ (vector of pLacZi), ABI4p-1::LacZ , ABI4p-2::LacZ , ABI4p-3::LacZ , and ABI4p-4::LacZ , and GAD itself, with ABI4p-4::LacZ , were co-transformed into the yeast strain EGY48 using standard transformation techniques. For the domain deletion assay, the GAD-DDT, GAD-PHD and GAD-(DDT+PHD) of PTM were co-transformed with ABI4p-4::LacZ into the yeast strain EGY48 using standard transformation techniques. Transformants were grown on proper dropout plates containing X-gal (5-bromo-4-chloro-3-indolyl-β- D -galactopyranoside) for blue colour development [42] . Protoplast transient expression assay The reporter construct ABI4p::Luc , the effector plasmid and the 35S::GUS construct were co-transformed into protoplasts [43] . After transformation, the protoplasts were incubated under light for 12–15 h. The protoplasts were pelleted and resuspended in 100 μl of 1× CCLR buffer (Promega). For the luciferase activity assay, 5 μl of the extract was mixed with 50 μl of luciferase assay substrate (Promega), and the activity was detected with the Modulus luminometer/fluorometer with a luminescence kit. For the GUS enzymatic assay, 5 μl of the extract was incubated with 50 μl 4-methylumbelliferyl β- D -glucuronide assay buffer (50 mM sodium phosphate, pH 7.0, 1 mM 4-methylumbelliferyl β- D -glucuronide, 10 mM EDTA, 10 mM β-mercaptoethanol, 0.1% sarkosyl, 0.1% Triton X-100) at 37 °C for 15 min, and the reaction was stopped by adding 945 μl of 0.2 M Na 2 CO 3 . The fluorescence was measured using a Modulus Luminometer/Fluorometer with a ultraviolet fluorescence optical kit (Turner Biosystems). The reporter gene expression levels were expressed as relative LUC/GUS ratios. Chromatin immunoprecipitation For immunoprecipitation, 10 μl of anti-H3K4me3, anti-H3K9,14ac (Upstate Biotechnology), or anti-PTM antibodies (rabbit antiserum against the synthesized peptides, Supplementary Table S1 ) were incubated in phosphate-buffered saline solution with Protein G-agarose (Upstate Biotechnology), and then 1 mg of chromatin protein extract was added. Finally, the purified DNA was diluted to 100 μl with 0.5 μl used for each PCR assay [44] . PCR primers used in the ChIP assays are described in Supplementary Table S2 . As negative controls, the ChIP experiments were performed using protein G-agarose with preimmune serum. Chloroplast isolation and fractionation The Arabidopsis leaves were homogenized in 330 mM sorbitol, 20 mM Tricin-NaOH, pH 7.6, 5 mM EGTA, 10 mM Na 2 CO 3 , 0.1% (w/v) bovine serum albumin (BSA) and 330 mg l −1 ascorbate, filtered and centrifuged for 5 min at 2,000 g . The pellet was resuspended in 330 mM sorbitol, 20 mM HEPES-KOH, pH 7.6, 5 mM MgCl 2 , 10 mM Na 2 CO 3 , 0.1% (w/v) BSA and 2.5 mM EDTA, and intact chloroplasts were isolated though a 40%/70% step Percoll gradient [45] . The intact chloroplasts were resuspended in hypertonic buffer (0.65 M sucrose, 10 mM Tricine-KOH, pH 7.9), and the suspension was homogenized in a Dounce tissue grinder. Thylakoids were then pelleted at 4,500 g for 30 min at 4 °C, and the crude envelopes were obtained after the supernatant was subjected to centrifugation at 200,000 g for 1 h. The crude envelopes were resuspended in 1 ml 0.4 M sucrose, 10 mM Tricine-KOH, pH 7.9, and then the suspension was concentrated through a discontinuous sucrose gradient (1, 0.8 and 0.46 M sucrose) at 120,000 g for 5 h. After centrifugation, the inner envelope and outer envelope fractions were recovered separately from the gradient, and the envelopes were further purified on linear sucrose gradients (0.59–1.2 M, 10 mM Tricine-KOH, pH 7.9) [46] . Isolation of nuclear protein extracts The nuclear protein extracts were isolated using the CelLytic PN Isolation/Extraction Kit (Sigma-Aldrich). Pull-down assays The pGST-PTM-PHD and the mutant proteins were expressed and purified using GST Bind Kits (Novagen) as described by the manufacturer's protocol. Biotinylated histone peptides (1 μg each; Supplementary Table S1 ) were incubated with 1 μg of purified pGST-PTM-PHD and the mutant proteins in binding buffer (0.1 M phosphate, 0.15 M NaCl, pH 7.2) overnight at 4 °C. After a 1-h incubation with Pierce Streptavidin Agarose Resin (Thermo Scientific), beads were washed five times with the binding buffer, and bound proteins were analysed by immunoblotting using an anti-GST antibody (Santa Cruz Biotechnology). Immunofluorescence microscopy The wild-type leaf sections were washed three times in PBS and incubated for 6 h at room temperature in a cell–wall digestion solution preheated at 37 ° C (20 mM MES, pH 5.7, 1.5% (w/v) cellulase R10, 0.4% (w/v) macerozyme R10, 0.4 M mannitol, 20 mM KCl, 10 mM CaCl 2 , 5 mM β-mercaptoethanol, 0.1% BSA, 1 mM phenylmethylsulfonyl fluoride). The protoplasts were washed twice in a solution of 2 mM MES, pH 5.7, 154 mM NaCl, 125 mM CaCl 2 and 5 mM KCl. For immunostaining, the protoplasts were treated with 0.05 μmol NF and 22 μg ml −1 Lin for 90 min in the presence or absence of CHX followed by fixation with 2% (w/v) paraformaldehyde for 15 min. Subsequently, the protoplasts were blocked with PBS (137 mM NaCl, 2.7 mM KCl, 10 mM Na 2 HPO 4 and 1.76 mM KH 2 PO 4 ) buffer containing 0.5% (w/v) BSA and 0.001% (v/v) Triton X-100 for 0.5 h and incubated with the anti-N-PTM antibodies in PBS-containing 0.1% (w/v) BSA for 4 h at 4 °C with very gentle shaking. The protoplasts were then washed three times in PBS-containing 0.005% (v/v) Triton X-100 (PBST) followed by a 2 h incubation with FITC-conjugated anti-rabbit secondary antibody (Molecular Probes; 1:200) in PBS-containing 0.5% (w/v) BSA at 4 °C with very gentle shaking. After three washes with PBST, the protoplasts were mounted on a glass slide in 50% (w/v) glycerol in Tris, pH 9.5, containing an antifade reagent (Bio-Rad) and 0.1 μg ml −1 4,6-diamidino-2-phenylindole [47] . Immunofluorescence was examined using a confocal laser scanning microscope (LSM510; Carl Zeiss). PTM processing For the HL treatment, 4-week-old detached Arabidopsis leaves, floating adaxial side up on water, were illuminated with a photon flux density of 1,600 μmol m −2 s −1 for various number of hours in the presence or absence of CHX. For treatments with NF and Lin, the Arabidopsis seedlings were grown in the 1/2 LS media in the presence of 220 μg ml −1 Lin and 5 μM NF. For treatments with protease inhibitors, pefabloc SC (4-(2-aminoethyl)-benzensulfonyl-flouride hydrochloride; 1 mg ml −1 , Roche) or pepstatin A (1 μg ml −1 , Sigma-Aldrich) was added under normal light condition for 1 h before HL treatments. How to cite this article: Sun, X. et al . A chloroplast envelope-bound PHD transcription factor mediates chloroplast signals to the nucleus. Nat. Commun. 2:477 doi: 10.1038/ncomms1486 (2011).